Crystal structures of wild type and disease mutant forms of the ryanodine receptor SPRY2 domain Ryanodine receptors (RyRs) form channels responsible for the release of Ca 2+ from the endoplasmic and sarcoplasmic reticulum. The SPRY2 domain in the skeletal muscle isoform (RyR1) has been proposed as a direct link with L-type calcium channels (Ca V 1.1), allowing for direct mechanical coupling between plasma membrane depolarization and Ca 2+ release. Here we present the crystal structures of the SPRY2 domain from RyR1 and RyR2 at 1.34–1.84 Å resolution. They form two antiparallel β sheets establishing a core, and four additional modules of which several are required for proper folding. A buried disease mutation, linked to hypertrophic cardiomyopathy and loss-of-function, induces local misfolding and strong destabilization. Isothermal titration calorimetry experiments negate the RyR1 SPRY2 domain as the major link with Ca V 1.1. Instead, docking into full-length RyR1 cryo-electron microscopy maps suggests that the SPRY2 domain forms a link between the N-terminal gating ring and the clamp region. Ryanodine receptors (RyRs) are membrane proteins responsible for the release of Ca 2+ from the endoplasmic and sarcoplasmic reticulum (ER/SR) [1] . Mammalian organisms contain three different isoforms (RyR1–3) [2] , [3] , [4] , [5] , [6] , with their expression profiles depending on the cell type. RyRs play major roles in excitation–contraction coupling, with RyR1 as the predominant form in skeletal muscle, and RyR2 in cardiac myocytes. These proteins represent the pinnacle of ion channel complexity: with molecular weights exceeding 2.2 MDa, they form docking sites for tens of auxiliary proteins and small molecules that can regulate their activities. Cryo-electron microscopy (cryo-EM) studies have shown that the RyRs form tetrameric assemblies that resemble the shape of a mushroom [7] , [8] , [9] , [10] : the stalk region is thought to traverse the membrane of the ER or SR, and the large cap is located entirely in the cytosol. The cap regulates the ability of the channel to open or close, turning RyRs into enormous allosteric membrane proteins [11] . A number of crystal structures have been reported, focusing mostly on the amino-terminal (N-terminal) three domains [12] , [13] , [14] , [15] , [16] , [17] , [18] , and a single domain containing a phosphorylation hot spot loop [19] , [20] . RyRs can be activated by Ca 2+ , the very same ion it permeates [21] , [22] . In cardiac myocytes, the triggering Ca 2+ primarily originates from the opening of L-type voltage-gated calcium channels located in the plasma membrane. In skeletal muscle, however, it has been shown that depolarization of the plasma membrane can trigger Ca 2+ release even in the absence of extracellular Ca 2+ . Many studies suggest that RyR1 and Ca V 1.1 form direct physical contacts, with Ca V 1.1 acting as the voltage sensor for RyR1 through direct mechanical coupling [23] , [24] , [25] , [26] , [27] . In addition, ‘retrograde’ signalling has been reported, whereby changes in RyR1 can affect the function of Ca V 1.1 (refs 28 , 29 ). Understanding how Ca V 1.1 and RyR1 can influence one another’s behaviour is one of the major puzzles in the field of excitation–contraction coupling. On the Ca V 1.1 side, several studies have shown the importance of the cytosolic loop connecting transmembrane repeats II and III (‘II–III loop’) [30] , [31] , [32] . Within RyR1, several regions of RyR1 that may bind this loop have been proposed through the use of pull-downs and chimeras between RyR1 and RyR2. Several interaction sites have been suggested [33] , [34] , [35] , [36] and a major focus has been on the SPRY2 domain [37] , [38] , [39] , [40] , [41] . SPRY domains lend their name to splA kinase and RyRs, where they were first identified. RyRs contain three such SPRY domains, conserved among vertebrates and invertebrates. Although they are founders for this family, no high-resolution structure has been reported for any of them. Here we describe the crystal structures of the SPRY2 domain of both RyR1 and RyR2, showing that they consist of additional modules not previously predicted. Their location in full-length RyR1 suggests a role for linking motions in the central gating ring, formed by the N-terminal domains, with the mobile corner region. We also analyse the effect of disease-causing mutations on the structure and stability. Overall structures of the RyR1 and RyR2 SPRY2 domains We solved the crystal structures of the SPRY2 domains of the two RyR isoforms, encoded by residues 1070–1246 in rabbit RyR1 and 1080–1253 in mouse RyR2. The RyR2 SPRY2 structure was solved via sulphur-SAD phasing, which was then used as a molecular replacement model for the RyR1 SPRY2 domain structure. The final resolutions were 1.84 Å (RyR1) and 1.34 Å (RyR2). Three molecules are present in the asymmetric unit for the RyR1 structure. As these are nearly identical ( Supplementary Fig. 1 ), we performed all analyses with chain A. 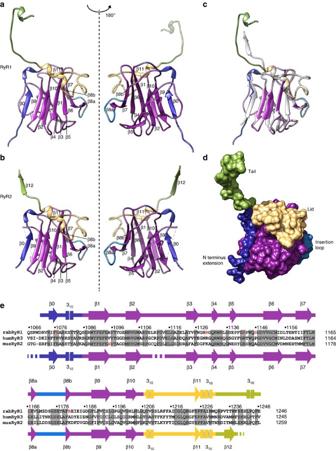Figure 1: Overall structure of the SPRY2 domain. (a) Two views of the RyR1 SPRY2 domain. Secondary structure elements are labelled. The core of the structure is shown in purple. Extra modules are shown in different colours (blue, N-terminal extension; yellow, lid; cyan, insertion loop; green, tail). (b) Two views of the RyR2 SPRY2 domain with colouring and labels as in panel A. (c) Superposition of the SPRY2 domains from RyR1 (colours) and RyR2 (grey). (d) Surface representation of the RyR1 SPRY2 domain with each module in a different colour, showing the extensive interactions between the modules. (e) Sequence alignment of the SPRY2 domains in RyR1, RyR2 and RyR3, with the secondary structures indicated. Colours represent the modules. Loop regions with structures are indicated by a solid line. Dotted lines represent parts of the construct that lack interpretable electron density. The red letters indicate positions of disease-causing mutations. Figure 1 shows the overall structures of the SPRY2 domains. It is immediately clear that these consist of several individual structural elements that make them substantially different from previously predicted SPRY2 domain structures. The core of the protein consists of a stretch of 10 β strands (β 1 –β 10 ), arranged in two antiparallel sheets, which was previously assumed to constitute the entire SPRY2 domain [38] , [40] , [42] . However, at the N terminus an extension is present, adding a supplementary beta strand (β 0 ) and a short 3 10 helix. A 10-residue loop (‘insertion loop’) is inserted in what is normally strand β 8 , splitting it up into two smaller strands β 8a and β 8b . Carboxyl-terminal (C-terminal) to the last β strand of the core is a region we named the ‘lid’, containing two 3 10 helices and a short β strand that forms β sheet interactions with the first strand of the core. The lid makes substantial hydrophobic interactions with both the N-terminal extension and the core, burying ~820 Å 2 of the surface area. The core, lid and insertion loop are in the exact same position in RyR1 and RyR2 ( Fig. 1c ). Because an identical arrangement is found in two structures for which the crystallization conditions and crystal contacts are entirely different, these arrangements appear stable and likely also occur in full-length RyRs. Figure 1: Overall structure of the SPRY2 domain. ( a ) Two views of the RyR1 SPRY2 domain. Secondary structure elements are labelled. The core of the structure is shown in purple. Extra modules are shown in different colours (blue, N-terminal extension; yellow, lid; cyan, insertion loop; green, tail). ( b ) Two views of the RyR2 SPRY2 domain with colouring and labels as in panel A. ( c ) Superposition of the SPRY2 domains from RyR1 (colours) and RyR2 (grey). ( d ) Surface representation of the RyR1 SPRY2 domain with each module in a different colour, showing the extensive interactions between the modules. ( e ) Sequence alignment of the SPRY2 domains in RyR1, RyR2 and RyR3, with the secondary structures indicated. Colours represent the modules. Loop regions with structures are indicated by a solid line. Dotted lines represent parts of the construct that lack interpretable electron density. The red letters indicate positions of disease-causing mutations. Full size image Immediately following this lid is an extended region (‘tail’). This unusual conformation in both structures is the direct result of crystal contacts ( Fig. 2a,b ). In both RyR1 and RyR2, the tail interacts with the same surface of a neighbouring molecule, although the orientation is different: parallel in RyR1, but forming an additional antiparallel β strand in RyR2. Despite these extensive crystal contacts, the constructs behave as monomeric species using size exclusion chromatography, suggesting that in solution the tail is more probable to form an intramolecular, rather than intermolecular interaction. Only the antiparallel arrangement can be formed, extending the antiparallel β sheet ( Fig. 2c ). A parallel intramolecular arrangement is sterically not allowed due to the limited length of the tail. The tail contains a Trp that forms extensive interactions and that is highly conserved among RyRs ( Supplementary Fig. 2 ). 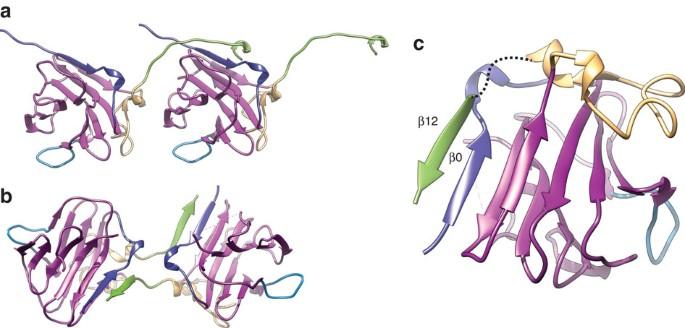Figure 2: Swapping of the tail region in the crystal lattice. Two neighbouring chains in the crystal lattice are shown for the SPRY2 domain of (a) RyR1 and (b) RyR2, indicating that the tail mediates crystal packing contacts with strand β0. In RyR2, the tail extends an antiparallel sheet. (c) Likely intramolecular arrangement for the tail in solution, shown here for the RyR2 SPRY2 domain. Figure 2: Swapping of the tail region in the crystal lattice. Two neighbouring chains in the crystal lattice are shown for the SPRY2 domain of ( a ) RyR1 and ( b ) RyR2, indicating that the tail mediates crystal packing contacts with strand β 0 . In RyR2, the tail extends an antiparallel sheet. ( c ) Likely intramolecular arrangement for the tail in solution, shown here for the RyR2 SPRY2 domain. Full size image In comparison with SPRY domains from other proteins, several elements appear unique to the SPRY2 domain ( Supplementary Fig. 3 ). The closest structural homologue is the SPRY domain from Ash2L, which also contains a ‘lid’, but still misses the insertion loop and contains two extra β sheets that replace the N-terminal and C-terminal extension strands. Two other SPRY domains are present within the RyR sequence. Both share low sequence identity with SPRY2 (~20%), and several insertions and deletions are present ( Supplementary Fig. 4 ). Neither of them seems to contain the insertion loop and the sequences within the additional modules are particularly dissimilar, suggesting that the three SPRY domains within RyRs have diverged substantially. Loss-of-function mutations in the RyR2 SPRY2 domain The SPRY2 domain of RYR2 harbours the position of a very unusual disease mutation (T1107M) that has been linked to hypertrophic cardiomyopathy [43] . Importantly, functional experiments have indicated a loss-of-function phenotype for the T1107M mutant, with a reduction in fractional Ca 2+ release and an increase in the threshold for its termination [44] . Since most mutations characterized in the cytosolic portions of RyRs are instead linked to gain-of-function phenotypes, we decided to take a closer look at this loss-of-function mutation. The corresponding residue in the mouse RyR2 (A1107) is buried, with the C β atom pointing towards a hydrophobic core ( Fig. 3a,c ). There is space for a Thr at this position, but a Met side chain would completely clash with Trp1156 ( Supplementary Fig. 5 ). Surprisingly, the A1107M mutation is tolerated within the individual domain, as indicated by the absence of any aggregation in size exclusion chromatography ( Supplementary Fig. 6 ). However, the substitution causes a significant destabilization of the domain, with the melting temperature decreasing ~9 °C compared with wild type ( Fig. 3b ). At a physiological temperature of 37 °C, ~22% of the domain is unfolded. Although the actual melting temperature will be different within full-length RyR2, where domain interactions may confer additional stability, there is a clear trend towards destabilization of the fold. 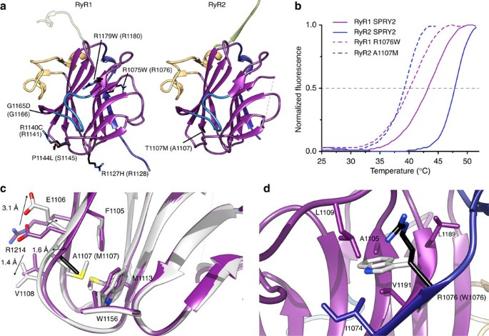Figure 3: Disease mutations. (a) Relative positions of disease-causing mutations (black sticks) in the RyR1 and RyR2 SPRY2 domains. Labels indicate the mutation in human RyRs, with the corresponding rabbit RyR1 and mouse RyR2 residue in brackets. (b) Thermal melting curves, as determined by thermofluor assays, for WT and mutant SPRY2 domains. The curves are the average of eight independent measurements. The obtained melting temperatures are (with s.d.): RyR1 SPRY2: 43.2±0.3 °C, RyR2 SPRY2: 47.9±0.3 °C, RyR1 R1076W: 40.2±0.5 °C, RyR2 A1107 M: 39.1±0.2 °C. (c) Close-up of the superposition of WT (colours) and A1107M SPRY2 (white) in RyR2. Ala1107 is shown in black. The arrows show the relative positional changes. These changes are best seen inSupplementary Movie S1. (d) Close-up of Arg1076 (black) in RyR1 SPRY2. A Trp side chain (white) at this site would cause a steric clash with neighbouring hydrophobic residues. Figure 3: Disease mutations. ( a ) Relative positions of disease-causing mutations (black sticks) in the RyR1 and RyR2 SPRY2 domains. Labels indicate the mutation in human RyRs, with the corresponding rabbit RyR1 and mouse RyR2 residue in brackets. ( b ) Thermal melting curves, as determined by thermofluor assays, for WT and mutant SPRY2 domains. The curves are the average of eight independent measurements. The obtained melting temperatures are (with s.d. ): RyR1 SPRY2: 43.2±0.3 °C, RyR2 SPRY2: 47.9±0.3 °C, RyR1 R1076W: 40.2±0.5 °C, RyR2 A1107 M: 39.1±0.2 °C. ( c ) Close-up of the superposition of WT (colours) and A1107M SPRY2 (white) in RyR2. Ala1107 is shown in black. The arrows show the relative positional changes. These changes are best seen in Supplementary Movie S1 . ( d ) Close-up of Arg1076 (black) in RyR1 SPRY2. A Trp side chain (white) at this site would cause a steric clash with neighbouring hydrophobic residues. Full size image We crystallized the corresponding A1107M mutant and solved its structure at 1.44 Å. The structural changes are best seen in a video that morphs between wild type and mutant ( Supplementary Movie 1 ). To allow the Met side chain to fit in the hydrophobic core, the backbone of residue 1107 is shifted over 1.6 Å. This shift now results in several changes at the surface. It affects the main chain positions of the neighbouring residues Glu1106 and Val1108, whose side chains adopt different conformations, resulting in positional shifts up to 3.1 Å ( Fig. 3c ). In the wild-type structure, Glu1106 forms a salt bridge with Arg1214, but in the mutant this salt bridge is lost and the electron density for the Arg1214 is absent, indicating that this residue has become flexible. In conclusion, the mutation induces a local misfolding resulting in surface changes at low temperatures, and has a substantial degree of unfolding at 37 °C. These combined effects likely underlie the loss-of-function phenotype associated with this mutation. Mutations in the RyR1 SPRY2 domain The RyR1 SPRY2 domain contains locations for five disease mutations ( Fig. 3a ). This includes R1075W (human numbering), identified in two patients from one family who died shortly after birth. Muscle biopsies indicated central core disease (CCD) [45] . The residue is strictly conserved, and is located at the end of the N-terminal extension strand (β 0 ), making multiple interactions with neighbouring residues. The stalk portion of the side chain is in hydrophobic contact with several hydrophobic residues ( Fig. 3d ), whereas the positively charged guanidinium group is exposed to the surface. In a model of the RyR1 SPRY2 domain where the tail is added in the antiparallel, intramolecular arrangement, the Arg1075 is also in contact with the tail ( Supplementary Fig. 7 ). Without substantial rearrangements, there would be no room for a bulkier Trp side chain, even in the absence of the tail strand. We tested the impact of the corresponding R1076W mutation in the rabbit RyR1 SPRY2 domain. The protein can still fold as it does not cause aggregation as measured by size exclusion chromatography ( Supplementary Fig. 6 ). However, thermofluor experiments show that the mutation destabilizes the domain reducing the melting temperature by ~3 °C ( Fig. 3b ). Although the effect on thermal stability is thus smaller than for the A1107M mutation in RyR2, the RyR1 SPRY2 domain is already less stable than in RyR2, and the melting temperature of the R1076W mutant SPRY2 is very similar to the RyR2 A1107M SPRY2. Our attempts to crystallize the mutant failed, suggesting that the structural rearrangements are substantial. On the basis of these observations, we predict that the human R1075W mutant may lead to a loss-of-function phenotype, consistent with CCD. Two other mutations in the RyR1 SPRY2 domain have also been identified in patients with CCD [46] . However, in both cases, an additional mutation was found, so the phenotype could be due to either one or their combination. The G1165D is located in a turn preceding strand β 8a in a region that interacts with the lid module ( Fig. 3a , Supplementary Fig. 8 ). An Asp residue at this position is expected to interfere with the interactions, as it would cause clashes with two hydrophobic residues of the lid ( Supplementary Fig. 8 ). The mutation is therefore highly likely to affect function of RyR1. In contrast with this, the R1179W mutation is exposed at the surface of the protein, and is thus not expected to interfere with folding ( Fig. 3a ). It can only be responsible for a disease phenotype if it is located at an interface with an auxiliary protein or another domain. In addition, two mutations in the SPRY2 domain have been linked to malignant hyperthermia (MH), a disorder linked to RyR1 gain of function [47] , [48] . The R1127H and R1140C mutations (human numbering) are both exposed at the surface of the protein ( Fig. 3a ). The substitutions are not predicted to create any steric hindrance, and therefore would only affect the surface properties of the domain. Similar to the R1179W mutation, they can only create a disease phenotype if they are located at an interface. Finally, the P1144L mutation was found in exome sequencing but it is unclear whether it is causative of MH [49] . Its corresponding residue is a Ser in the rabbit RyR1 sequence, and is exposed at the surface. To consider the further impact of these disease mutations, we explored the potential role of the SPRY2 domain by analysing its proposed binding and its location in full-length RyRs. Interaction with the Ca V 1.1 II–III loop Several studies have supported a role for the RyR1 SPRY2 domain in direct interactions with the cytosolic II–III loop of Ca V 1.1. With a very soluble and well-behaved RyR1 SPRY2 domain in hand, we tested its ability to bind the II–III loop using isothermal titration calorimetry (ITC). However, even at high concentrations, the heat signals were indistinguishable from background titrations ( Fig. 4a ), indicating that any binding between the two, if at all, would be extremely weak ( K d >1 mM). 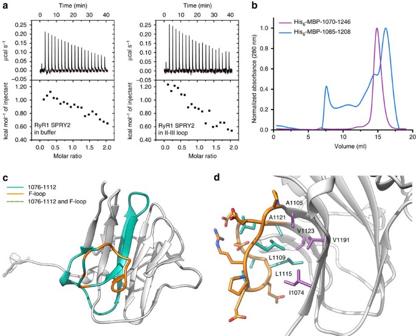Figure 4: Absence of interactions between the RyR1 SPRY2 domain and the CaV1.1 II–III loop. (a) Raw ITC data comparing the titrations of RyR1 SPRY2 (887 μM) into buffer or the II–III loop (89 μM), showing no significant difference in heat signals. (b) Size exclusion chromatograms (analytical Superdex200) of MBP fusions of RyR1 1070–1246 and 1085–1208. Removal of the MBP tag from the 1085–1208 construct led to complete loss of the protein. (c) Structure of the RyR1 SPRY2 domain, highlighting residues 1076–1112 (human numbering, green) and the ‘F-loop’, encoded by residues 1107–1121 (human numbering, orange). Alternating colours show regions of overlap. Both are involved in extensive interactions with the remainder of the domain and are unlikely to adopt a native conformation in isolation. (d) Detail of the RyR1 F-loop (orange), indicating its hydrophobic side chains in green sticks. These interact extensively with hydrophobic residues on the rest of the SPRY2 domain (purple sticks). Figure 4: Absence of interactions between the RyR1 SPRY2 domain and the Ca V 1.1 II–III loop. ( a ) Raw ITC data comparing the titrations of RyR1 SPRY2 (887 μM) into buffer or the II–III loop (89 μM), showing no significant difference in heat signals. ( b ) Size exclusion chromatograms (analytical Superdex200) of MBP fusions of RyR1 1070–1246 and 1085–1208. Removal of the MBP tag from the 1085–1208 construct led to complete loss of the protein. ( c ) Structure of the RyR1 SPRY2 domain, highlighting residues 1076–1112 (human numbering, green) and the ‘F-loop’, encoded by residues 1107–1121 (human numbering, orange). Alternating colours show regions of overlap. Both are involved in extensive interactions with the remainder of the domain and are unlikely to adopt a native conformation in isolation. ( d ) Detail of the RyR1 F-loop (orange), indicating its hydrophobic side chains in green sticks. These interact extensively with hydrophobic residues on the rest of the SPRY2 domain (purple sticks). Full size image Previous biochemical experiments were performed using only the ‘core’ of the SPRY2 domain, consisting of residues 1085–1208 in RyR1 (refs 37 , 38 , 39 ). This represents the major module in the structure, but on expression and purification of such a construct it proved to be poorly soluble and caused major aggregation as indicated by size exclusion chromatography ( Fig. 4b ). This aggregation is observed even despite the presence of a stabilizing maltose-binding protein (MBP) fused at the N terminus. Proteolytic removal of the MBP (see Methods) caused complete loss of the protein. Even constructs in which only the N-terminal extension or lid was deleted separately already appeared to be misfolded. This is in agreement with the extensive amount of hydrophobic surface that is buried by these extra modules. As such, any previous studies using only the SPRY2 core or portions thereof are likely to yield unfortunate false positives because these missed major elements required for stability of the SPRY2 domain. We conclude that the RyR1 SPRY2 domain is unlikely to be a major determinant of the RyR1–Ca V 1.1 interaction. As a result, the disease-causing mutations also are unlikely to affect binding to Ca V 1.1 directly. We next explored a possible role for the SPRY2 domain by analyzing its location. Location of the SPRY2 domain in full-length RyR1 We attempted to locate the position of the RyR1 SPRY2 domain in available cryo-EM maps of full-length RyR1. We used an unbiased approach, employing systematic six-dimensional searches (three rotational and three translational parameters) as implemented in Situs [50] . We analysed and ranked the cross-correlation coefficients for each of the tested locations. As noted before, the addition of a Laplacian filter appeared crucial to obtain sensible docking results [12] . In three of the tested maps (EMDB accession numbers 5014,1606, and 1607) [8] , [9] , the top hit consistently docked to the same location and, reassuringly, in the same orientation ( Fig. 5a ). Plotting the correlation coefficients of the top hits shows that there is some contrast, especially in the EMD5014 map where the top hit is separated by the mean of the next nine hits by up to ~8 s.d. 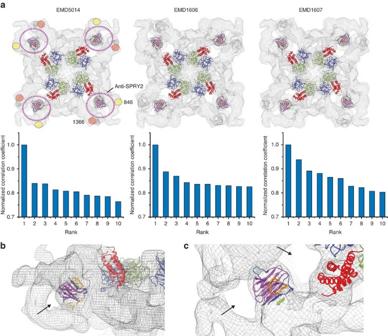Figure 5: Location of the SPRY2 domain in intact RyR1. (a) Top docking solutions for the RyR1 SPRY2 domain in three different cryo-EM maps of full-length RyR1. The colours for the SPRY2 domain are as inFig. 1. The positions of the N-terminal three domains (blue, green, red) are also shown for reference. The bar graphs below show the normalized correlation coefficients for the top 10 unique hits in each map. Due to the four-fold symmetry, each solution comes up four times, but is only shown once in the bar graphs. The filled circles in the top left panel represent the locations for difference density observed for RyR2-GFP insertions near RyR2 residues 846 (yellow circle)53and 1366 (orange circle)52. The purple dotted circle represents the area where difference densities were observed for cryo-EM studies of anti-SPRY2 antibody bound to RyR1 (ref.42). (b) ‘Side view’ of the docked SPRY2 domain, showing its solvent accessibility at the periphery of the RyR (arrow). (c) Close-up showing that two-solvent channels (arrows) line the docked SPRY2. The loop encoded by residues 1107–1121 is shown in orange. It is accessible from both solvent channels. Figure 5: Location of the SPRY2 domain in intact RyR1. ( a ) Top docking solutions for the RyR1 SPRY2 domain in three different cryo-EM maps of full-length RyR1. The colours for the SPRY2 domain are as in Fig. 1 . The positions of the N-terminal three domains (blue, green, red) are also shown for reference. The bar graphs below show the normalized correlation coefficients for the top 10 unique hits in each map. Due to the four-fold symmetry, each solution comes up four times, but is only shown once in the bar graphs. The filled circles in the top left panel represent the locations for difference density observed for RyR2-GFP insertions near RyR2 residues 846 (yellow circle) [53] and 1366 (orange circle) [52] . The purple dotted circle represents the area where difference densities were observed for cryo-EM studies of anti-SPRY2 antibody bound to RyR1 (ref. 42 ). ( b ) ‘Side view’ of the docked SPRY2 domain, showing its solvent accessibility at the periphery of the RyR (arrow). ( c ) Close-up showing that two-solvent channels (arrows) line the docked SPRY2. The loop encoded by residues 1107–1121 is shown in orange. It is accessible from both solvent channels. Full size image Searches in a fourth map (EMDB 1275) only yielded nonsense positions, such as the column positions, transmembrane area and the position where the N-terminal area was found to be located [12] , [14] , [51] . As expected with nonsense solutions, there was no contrast between the top hit and the following solutions ( Supplementary Fig. 9 ). Because there are two other SPRY domains within the RyR polypeptide, there is the inherent possibility that the top hit could correspond to either SPRY1 or SPRY3. In the absence of crystal structures for these, this cannot be formally tested, but docking of homology models in the EMDB 5014 map yielded entirely different positions. In addition, docking of other known SPRY structures also yielded different positions, suggesting that there is sufficient resolution in the maps to discriminate between proteins of the same fold. We therefore propose the location shown in Fig. 5 as the most likely position for the SPRY2 domain. This setting is strategically located between the corner, an area shown to undergo large conformational changes during opening and closing [9] , and the central rim, formed by the N-terminal three domains establishing a ‘gating ring’ that is thought to modulate channel open probability [11] , [14] . The SPRY2 domain is likely required to couple the conformational changes in both areas, and disease-causing mutations on its surface may interfere with this process. Importantly, this location is in agreement with several previous studies. First, several antibodies raised against RyR1 SPRY2 have been shown to access their epitopes in native, folded RyR1 (ref. 42 ). In the proposed dock, the SPRY2 domain is accessible via two solvent channels and from the periphery ( Fig. 5b,c ). Cryo-EM reconstructions of antibody-bound complexes showed difference density in the clamp region, in an area compatible with our proposed SPRY2 position, especially given the ~160 Å dimensions of antibodies ( Fig. 5a , left panel, dotted circles). One of the antibodies was raised against residues 1107–1121, and this loop is accessible via two-solvent channels. Second, several cryo-EM studies have been performed on green fluorescent protein (GFP) fusions of RyR2. In one of these, GFP was inserted after RyR2 residue Thr1366, ~110 residues downstream of the SPRY2 sequence, and difference density was shown in subregion 6 (ref. 52 ) Another study inserted GFP near residue Tyr846, ~200 residues upstream of the SPRY2 domain, yielding difference density in the top portion of subregion 9 (ref. 53 ) So although no GFP insertion studies have been reported for the SPRY2 domain, insertion studies in the neighbouring domains within the sequence appear compatible with the proposed SPRY2 position, which is located directly in between these two difference densities ( Fig. 5a , left panel). A recent fluorescence resonance energy transfer (FRET) study using an insertion at position 1358, downstream of the SPRY2 domain, also yields a position compatible with our proposed SPRY2 location [54] . The RyR is a large allosteric membrane protein. Thanks to the presence of multiple domains located in the cytosolic cap, this membrane protein giant can receive input from tens of proteins and small molecules. One type of domain, the so-called ‘SPRY’ domain, is repeated three times in the RyR sequence [1] , and these are conserved from mammalian species all the way down to Drosophila and C. elegans. However, up to now, no structure from any SPRY domain of any RyR had been reported. Here we show high-resolution crystal structures of the SPRY2 domain of both RyR1 and RyR2. Contrary to previous predictions, this domain consists of several distinct modules (N-terminal extension, lid, insertion loop and tail) that add to what was previously thought to contain the SPRY2 domain. At least two of these modules, the N-terminal extension and lid, are absolutely required for proper folding of the domain. RyRs are the target for disease-causing mutations that mostly result in MH [55] or CCD [56] for RyR1 or in catecholaminergic polymorphic ventricular tachycardia [57] for RyR2. A common theme is that most mutations on the cytosolic cap have been linked to a gain of function, resulting in premature or prolonged release of Ca 2+ into the cytosol. The SPRY2 structures allowed us to map six mutations. Interestingly, they segregate into two groups, with three mutations either fully or partially buried within the domain, and three fully exposed at the surface. The buried T1107M mutation targets RyR2 and has been linked to hypertrophic cardiomyopathy [43] , as well as CPVT [58] . It is unclear how it could result in two different phenotypes, but functional experiments have clearly shown it to confer a rare loss-of-function phenotype with early termination of Ca 2+ release [44] . The mutation causes a significant thermal destabilization, resulting in 22% unfolding at physiological temperatures. In addition, it induces local misfolding, which results in conformational changes at the surface. Although the folding in intact RyR2 can be stabilized through domain–domain interactions, the 9 °C shift in melting temperature stability suggests a trend towards significant destabilization, suggesting that misfolding of the SPRY2 domain may generally lead to loss-of-function phenotypes. Two RyR1 mutations (G1165D, R1075W) also affect partially buried residues. Interestingly, both of them have been linked to CCD, a disorder that can be associated with loss-of-function phenotypes in RyR1. Although both mutations were also found in conjunction with mutations elsewhere in RyR1, we predict they interfere with proper folding and either contribute or are fully responsible for the disease phenotype. Three other mutations are found at the surface. Two of these have been linked to MH, a disorder characterized by gain-of-function of RyR1, and another has been linked to CCD. Since CCD can be linked to both gain and loss of function, a possible interpretation here is that mutations interfering with folding of SPRY2 create loss-of-function, whereas mutations on the surface create gain-of-function phenotypes. For the three mutations at the surface to be disease causing, they have to lie at an interface with an auxiliary protein or other domain. To identify what this might be, we analysed its interaction with a proposed binding partner and its location in full-length RyR. In the absence of a high-resolution structure, it was previously assumed that the SPRY2 domain only consisted of a smaller region, encoded by human RyR1 residues 1085–1208. However, it is now clear that the SPRY2 domain consists of additional portions that add ~43% of extra sequence, and our data show that the shorter construct causes aggregation, in stark contrast with the high solubility and monomeric nature of the crystallized 1070–1246 construct. In the presence of these additional modules, our ITC experiments fail to recapitulate the interaction with the Ca V 1.1 II–III loop, indicating that the SPRY2 domain cannot be the major determinant of the RyR1–Ca V 1.1 interaction. Previous experiments also suggested that an even smaller portion of the SPRY2 domain, encoded by residues 1076–1112, could bind to the II–III loop [41] . However, it is clear from the structure that such a fragment would not be able to fold in its native conformation, as it isolates single β strands from two different β sheets ( Fig. 4c ). Other experiments have further narrowed down the interaction to a loop encoded by residues 1107–1121, and showed that this peptide, in isolation, can affect the activity of RyR1 in planar lipid bilayers [40] . However, it is clear that this loop, which previously was thought to be extended [38] , makes substantial interactions with the remainder of the structure, burying hydrophobic side chains ( Fig. 4d ). The loop is highly unlikely to be adopting this stabilized conformation in isolation. Most likely, the interactions between RyR1 and Ca v 1.1, whether direct or via an intermediate protein, involve one or multiple RyR1 segments that have previously been suggested to be important for E–C coupling [32] , [33] , [34] , [35] . A popular method for studying RyR structure function is the use of isolated RyR peptides and to measure their effect on RyR function. It was shown that the ‘F-loop’, encoded by RyR1 residues 1107–1121, could increase the activity of RyR1 in planar lipid bilayers [40] . However, this loop forms extensive hydrophobic interactions with the remainder of the SPRY2 domain ( Fig. 4d ), and is thus very unlikely to adopt a native structure in isolation. It is unclear then why such a peptide could cause a functional effect. The same is true for a peptide in the N-terminal region of RyR2 (residues 163–195), which was shown to increase leak of Ca 2+ through RyR2 (ref. 59 ), but is largely an integral part of the β-trefoil core of domain A [15] , [16] , showing that it is impossible to adopt the same conformation in isolation. It may simply be that RyRs are sensitive to several unfolded peptides that do not necessarily mimic a native structure found in intact RyRs. Obtaining a high-resolution structure of the entire RyR has thus far been unsuccessful. The next best thing is to obtain high-resolution structures of individual domains or domain clusters, and then to locate these by finding the best position in full-length RyR cryo-EM maps. RyR1 reconstructions are available in the 10–12 Å range [7] , [8] , [9] , [60] , and these have allowed locating the N-terminal three domains of RyR1 with high accuracy to the central rim [12] , [14] . Thanks to the larger size, locating a three-domain structure appeared straightforward, with high contrast between the correlation coefficient of the top hit compared to the next hits in the ranking. The position of the N-terminal region was also confirmed via the difference cryo-EM and FRET measurements [51] . However, with single-domain structures, the contrast is typically lower [19] . Locating the SPRY2 domain yielded consistent results among three out of four RyR1 cryo-EM maps ( Fig. 5a ). Given that the refined positions appear to adopt the exact same relative orientation of the domain in all three maps, we propose this location as the most likely site for the SPRY2 domain. There is currently no report of any cryo-EM study using the SPRY2 domain as a position for insertions. However, the proposed location of the SPRY2 domain is in agreement with previous cryo-EM studies, which used insertions of GFP ~200 residues upstream [53] or ~110 residues downstream [52] of the SPRY2 domain. The proposed location of SPRY2 is directly in between the two difference densities ( Fig. 5a , left panel). In addition, cryo-EM reconstructions of RyR1 bound to antibodies raised against the SPRY2 domain are also consistent with this location [42] . One antibody was raised against the ‘F-loop’, which is accessible in the docked SPRY2 via two solvent channels. However, some structural changes may be necessary to allow access to the antibodies, which may explain why most of the RyR1 particles did not have antibodies bound to each subunit simultaneously [42] . Interestingly, antibodies raised against the SPRY2 domain were found to increase RyR1 activity in planar lipid bilayers, which would be expected if conformational changes are required for antibody binding. Importantly, this location is directly in between the corner region and the central rim. Both areas have been shown to undergo large conformational changes during channel opening [9] , [14] . The N-terminal three domains have been shown to form a ring near the four-fold symmetry axis [12] , and opening of the channel is coupled to disruption of an intersubunit interface [14] . The corner positions have been shown to move ‘downward’ towards the SR membrane during channel opening [9] . The SPRY2 domain, together with other domains, is likely involved in linking these transitions and the disease-causing mutations may then interfere with this process. One of the contacts seems to involve the insertion loop, a loop that cuts strand β8 normally found in canonical SPRY folds, into two smaller strands. Interestingly, two of the mutations located at the surface (R1179W, R1140C) flank this loop, and may thus interfere directly with this domain–domain interaction. The identities of the domains directly contacting SPRY2 remain to be found. Importantly, the RyR sequence contains two additional predicted SPRY domains. Homology models for these domains did not dock to the proposed SPRY2 location, which is not surprising given their low amount of sequence identity with SPRY2 (~20%) and the multiple insertions and deletions ( Supplementary Fig. 4 ). Similarly, we have previously shown that the cryo-EM maps can discriminate between domains A and B, which both form β-trefoil folds with twelve β strands each [12] . Despite the same fold, and a near perfect superposition of the β strands, the overall shape is largely determined by the loop regions of these domains, which determines their docked location. To further confirm the SPRY2 location, FRET experiments and further difference cryo-EM studies will be invaluable for experimental verification and to suggest possible interacting domains. Expression, purification and crystallization Rabbit RyR1 (1070–1246, 1085–1208) and mouse RyR2 (1080–1253) were cloned into the pET28 HMT vector [16] . Mutations were introduced by the Quikchange method (Stratagene). Human Ca V 1.1 II–III loop (666–787) was cloned in a pET24a vector containing a C-terminal hexahistidine tag using NdeI and XhoI restriction sites. At the N terminus, MBP was attached along with a tobacco etch virus (TEV) protease cleavage site. Cultures were grown in 2 × YT broth to an OD 600 ~0.8–1 at 37 °C. The temperature was then lowered to 18 °C, cells were induced with 0.2 mM isopropyl-β- D -thiogalactoside and allowed to grow for a total of 22–24 h. Cell pellets (2 l)were frozen at −20 °C. Cell pellets were lysed by sonication after addition of 5 ml glycerol, 40 ml Buffer A (250 mM KCl, 10 mM HEPES 7.4) supplemented with 25 μg ml −1 DNase I, 25 μg ml −1 lysozyme, 1 mM PMSF and 10 mM β-mercaptoethanol (bME). The lysate was centrifuged for 30 min at 35,000 g and a clarified supernatant was loaded onto a PorosMC (Tosoh Biosep) or TALON (GE Healthcare) column. The column was washed with 5–10 column volumes (CVs) of Buffer A followed by 5 CV of 2% Buffer B (250 mM KCl, 500 mM imidazole pH 7.4). The 2% Buffer B wash was omitted for all RyR2 constructs. Protein was eluted with 30% Buffer B, TEV protease added and immediately placed in a dialysis containing Buffer A at room temperature for 4 h or overnight. TEV protease was removed by loading the cleavage mixture onto a second PorosMC or Talon column with the flow-through collected. Excess MBP was removed by passing the flow-through over an amylose column. The flow-through was diluted threefold and further purified by anion-exchange chromatography with a Hiload-Q (GE Healthcare) equilibrated with Buffer C (20 mM HEPES pH 7.4) then on a gradient from 15–30% Buffer D (1M KCl, 20 mM HEPES pH 7.4) over 12 CVs. The protein was concentrated and polished by gel-filtration chromatography on a Superdex 200 (GE Healthcare). Protein crystals were grown by the hanging-drop method at 4 °C for RyR1 and at room temperature for RyR2. RyR1 SPRY2 domain (5–10 mg ml −1 ) was crystallized in 0.9–1.1 M sodium citrate pH 6.5. RyR2 SPRY2 domain (4 mg ml −1 ) and its mutant were crystallized in 0.2 M sodium formate, 18–25% PEG3350. Data collection and structure determination Crystals were harvested and flash-frozen in solutions containing the original growth conditions supplemented with 30% glycerol (RyR1) or 25% isopropyl alcohol (RyR2). Diffraction data were collected at the Canadian Light Source beamline 08ID-1 and the Advanced Photon Source beamline 23-ID-D-GM/CA. Data were processed with XDS [61] . Initial phases were calculated by Sulfur-SAD with Autosol [62] using native sulfur atoms on the RyR2 SPRY2 WT structure collected at 6.5 keV. The initial structure was further refined against a 1.34 Å data set using PHENIX [63] and manual model building using COOT [64] . The RyR2 SPRY2 structure was used as a search model for molecular replacement to solve the RyR1 structure and RyR2 SPRY2 A1107M mutant. Typical electron density is shown in Supplementary Fig. 10 . Table 1 contains the statistics for data collection and refinement. Coordinates and structure factors for all described structures are available in the Protein Data Bank with accession codes 4P9I, 4P9J, 4P9L. Table 1 Data collection and refinement statistics. Full size table Cryo-EM docking The ‘colores’ programme in the SITUS suite [50] was used to dock the RyR1 SPRY2 domain, containing the C-terminal tail in the antiparallel configuration, into four different RyR1 cryo-EM maps with EMDB entries 1606, 1607, 1275 and 5014. Six-dimensional searches were performed with a rotational sampling of 3° and with off-lattice Powell optimization. No density cutoff was applied and a Laplacian filter was used throughout. Thermofluor thermal shift assays Protein stability was measured by fluorescence [16] , [65] . Protein (10 μl; 1.5 mg ml −1 ) was mixed with 5 μl of a 1/500 dilution of SYPRO orange (Invitrogen) and diluted to 50 μl with buffer (150 mM KCl, 10 mM sodium phosphate pH 7.4, 14.3 mM bME). Thermal melts were performed eight fold using a DNA Engine Opticon 2 real-time PCR machine (Biorad) with the SYBR green filter. The temperature was increased from 25 °C to 95 °C in 0.5 °C increments with each step held constant for 15 s. Curves were normalized and the midpoints were taken as the melting points. ITC Proteins were dialyzed against 150 mM KCl, 10 mM HEPES (pH 7.4), 10 mM bME and 1 mM NaN 3 at 4 °C. Concentrations were determined by the method of Edelhoch [66] . Titrations consisted of 20 injections of 2 μl RyR1 SPRY2 domain into the cell containing either buffer or II–III loop. Concentrations used are noted in the figure legends. Experiments were performed at 25 °C and a stirring speed of 1,000 r.p.m. on an ITC200 instrument (GE Healthcare). All data were processed using Origin 7.0. Accession codes : Coordinates and structure factors for all described structures are available in the Protein Data Bank with accession codes 4P9I , 4P9J , 4P9L . How to cite this article : Lau, K. et al. Crystal structures of wild type and disease mutant forms of the Ryanodine receptor SPRY2 domain. Nat. Commun. 5:5397 doi: 10.1038/ncomms6397 (2014).